TargetingMycobacterium tuberculosisnucleoid-associated protein HU with structure-based inhibitors The nucleoid-associated protein HU plays an important role in maintenance of chromosomal architecture and in global regulation of DNA transactions in bacteria. Although HU is essential for growth in Mycobacterium tuberculosis (Mtb), there have been no reported attempts to perturb HU function with small molecules. Here we report the crystal structure of the N-terminal domain of HU from Mtb. We identify a core region within the HU–DNA interface that can be targeted using stilbene derivatives. These small molecules specifically inhibit HU–DNA binding, disrupt nucleoid architecture and reduce Mtb growth. The stilbene inhibitors induce gene expression changes in Mtb that resemble those induced by HU deficiency. Our results indicate that HU is a potential target for the development of therapies against tuberculosis. In bacteria, nucleoid-associated proteins (NAPs) represent a prominent group of global regulators that control genome compaction, chromosomal architecture and various DNA transactions such as, replication, transcription, recombination and repair [1] , [2] , [3] , [4] , [5] . HU, a small dimeric protein, is a key NAP in eubacteria [6] , [7] . In Escherichia coli , the function of HU as a global regulator of transcription is established by its control over 353 genes comprising 229 operons [8] . Mutation and gene disruption analyses have validated HU’s importance across species. The hupAB double mutant of E. coli shows slow growth and a highly pleotropic phenotype [9] , [10] , while in Bacillus subtilis , mutation in HU is lethal [11] . Over the ages of human history, Mtb has remained a formidable pathogen [12] claiming millions of lives. With 8.7 million new cases, 1.45 million deaths in 2011 alone [13] , and emergence of multidrug-resistant tuberculosis (TB) [14] , Mtb has re-emerged as an enormous challenge to public health system worldwide. Moreover, TB and HIV co-infection [15] , and the appearance of extensively drug-resistant TB [16] have necessitated intense on-going search for novel drug targets [17] and new drugs [18] . Exploration through high-density mutagenesis and deep sequencing [19] , [20] for defining the genes required for growth has identified hupB (HU-coding gene; gene id: 15610123) to be essential to Mtb. Despite its importance in Mtb, there has not been any attempt so far to identify molecules that target MtbHU and perturb its function. This is presumably due to the general perception that large and adaptive interfaces, such as the DNA-binding surface of HU, are not ‘ligandable’ [21] , making HU a challenging target. The present study is envisaged to fill the lacunae, and to develop strategies to target NAPs in general. Here we report the X-ray crystal structures of two polymorphs of the N-terminal domain of MtbHU (MtbHU N ) at 2.04 and 2.48 Å resolutions. The ‘core’ of the MtbHU–DNA interaction interface is identified. Docking analysis with the interaction core, and various biochemical, biophysical, mutational and biological studies show that two trans -stilbene derivatives [22] , [23] inhibit MtbHU binding to DNA. Furthermore, these compounds perturb the nucleoid architecture and curtail Mtb growth, indicating that HU can be targeted. The expression of a common set of genes is downregulated to a similar extent in a conditional MtbHU knockdown strain and in inhibitor-treated cells. Our work indicates that important NAPs such as HU in Mtb are likely to be ‘druggable’, creating opportunities for the design of new antimicrobials. Crystallization of MtbHU MtbHU (Swiss-Prot ID: P95109) contains two distinct domains. The N-terminal domain (MtbHU N ) is highly conserved among the members of Mycobacterium and Actinomyces . The C-terminal domain consists of degenerate sequence motifs of Lys, Ala and Pro rich repeats resembling eukaryotic histone H1. Studies with Mycobacterium smegmatis HU suggest that C-terminal extension may play a role in DNA protection and compaction [6] . Sequence comparison revealed 86–100% identity within the N-terminal region of HU, establishing MtbHU N as a prototypic molecule for various pathogens including M. tuberculosis , M. leprae , M. bovis and Nocardia ( Supplementary Fig. 1 ). We cloned the Mtb hupB , overexpressed and purified the recombinant MtbHU from E. coli BL21 cells to near homogeneity (Methods; Supplementary Fig. 2a ). Plate-shaped monoclinic crystals, belonging to P2 1 and P2 space groups, were obtained using hanging drop vapour diffusion method. The X-ray crystal structure of MtbHU N homodimer was determined at 2.04 and 2.48 Å resolutions for the two different crystal forms. Refined structures (see Methods for details) of MtbHU N have been deposited in protein data bank with Ids 4PT4 and 4DKY. 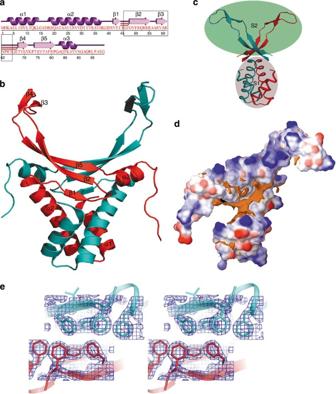Figure 1: Overview of MtbHUNdimer crystal structure. (a) MtbHUN(residues 1–99) sequence with secondary structural elements; boxed sequence spanning residues 46–65 corresponds to the Prosite pattern PS00045, common to HU-IHF fold. (b) The crystal structure of MtbHUNdimer (protomer A coloured red; protomer B coloured teal) is shown in cartoon representation. In the dimer, helices α1, α2 assemble to form a four-helix bundle, while β2, β3, β4 and β5 define a DNA-binding β cleft. (c) MtbHUNdimer can be divided into two subdomains, S1 consisting of the four helix bundle and S2 containing the DNA-binding cleft. (d) The MtbHUNprotomer dimerizes through the collapse of large hydrophobic patches at the interface. The surface profile of MtbHUNis generated with colour codes corresponding to surface electrostatic and hydrophobicity; Blue: positive, red: negative, orange: hydrophobic). (e) The base of S2, formed by anti-parallel β-sheet regions is stabilized by aromatic cluster of eight Phe rings (Phe47, 50, 79 and 85) from two protomers. 2Fo−Fc electron density map of aromatic cluster is contoured at 1.5σlevel and displayed in stereo image representation with side chains as sticks. Data statistics are given in Table 1 . Table 1 Data collection and refinement statistics. Full size table Structural overview Each protomer of MtbHU N is sequentially made up of two α-helices, α1 and α2, followed by five β-strands numbered β1 to β5, that are anti-parallel in arrangement and finally terminates in a short α-helix, α3 ( Fig. 1a , residues 1–99). Two such protomers wrap around each other to form a dimeric functional unit, giving rise to the ‘HU-IHF fold’ ( Fig. 1b ) [24] , [25] . Figure 1: Overview of MtbHU N dimer crystal structure. ( a ) MtbHU N (residues 1–99) sequence with secondary structural elements; boxed sequence spanning residues 46–65 corresponds to the Prosite pattern PS00045, common to HU-IHF fold. ( b ) The crystal structure of MtbHU N dimer (protomer A coloured red; protomer B coloured teal) is shown in cartoon representation. In the dimer, helices α1, α2 assemble to form a four-helix bundle, while β2, β3, β4 and β5 define a DNA-binding β cleft. ( c ) MtbHU N dimer can be divided into two subdomains, S1 consisting of the four helix bundle and S2 containing the DNA-binding cleft. ( d ) The MtbHU N protomer dimerizes through the collapse of large hydrophobic patches at the interface. The surface profile of MtbHU N is generated with colour codes corresponding to surface electrostatic and hydrophobicity; Blue: positive, red: negative, orange: hydrophobic). ( e ) The base of S2, formed by anti-parallel β-sheet regions is stabilized by aromatic cluster of eight Phe rings (Phe47, 50, 79 and 85) from two protomers. 2Fo−Fc electron density map of aromatic cluster is contoured at 1.5 σ level and displayed in stereo image representation with side chains as sticks. Full size image The fold is characterized by two subdomains, the α-helical dimerization domain (S1), which resembles pillars, on which the β-sheet dimerization domain, that is, the DNA-binding domain (S2), rests. The S1 domain is a four-helix bundle formed by α1 and α2 from each protomer. The S2 domain is a β-saddle, whose base is formed by β2 and β5 of each protomer, and the arms formed by β3, β4 and the intervening loops ( Fig. 1c ). Dimerization results in the burial of a large surface (4,360 Å 2 ; Fig. 1d ), with an energy of assembly dissociation Δ G diss =32.1 kcal mol −1 (calculated by PISA [26] for 4PT4), resulting in a stable MtbHU homodimer, the functional unit of the protein. At the bottom of the β-saddle is a cluster of Phe rings, viz., Phe47, Phe50, Phe79 and Phe85, contributed by each protomer to form the aromatic cluster ( Fig. 1e ). The homodimeric nature was evident from glutaraldehyde-mediated crosslinking studies (Methods; Supplementary Fig. 2b ). The quantity of the cross-linked dimeric species increased with higher concentrations of glutaraldehyde. The asymmetric unit of each crystal form contains two protomers of HU, independent of the crystallographic symmetry, and this allowed us to compare and examine the structures of the MtbHU N protomers, captured in different crystallographic environments. Superposition of main chain N, Cα and C atoms of the MtbHU N protomers showed a r.m.s.d. (root mean square deviation) of 1.2–2.5 Å in the stretch of residues from 54 to 75 ( Supplementary Fig. 3a,b ), whereas the average r.m.s.d. for the structure is ~0.5 Å. Distribution of average isotropic displacement parameters derived from the crystallographic B-factors also indicated that this region is structurally mobile ( Supplementary Fig. 3c ). The HingeProt server [27] and Translation/Libration/Screw motion determination (TLSMD) [28] both predicted that residues 54–75 in MtbHU are dynamic, whereas residues 1–54 and 75–99 constitute the relatively rigid parts ( Supplementary Methods and Supplementary Fig. 3d,e ). The structural flexibility of MtbHU’s DNA-binding domain may have implications in binding and bending various kinds of DNA, and is therefore important for its function as a nucleoid architectural protein. 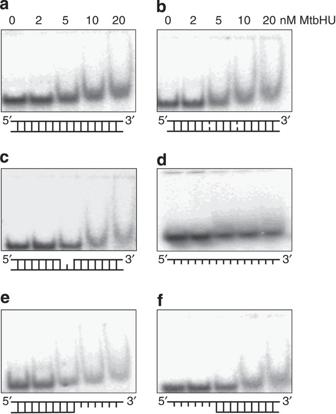Figure 2: Binding of MtbHU to different DNA substrates. (a–f) Comparative EMSA showing the binding of increasing amounts of MtbHU to a fixed concentration of different DNA substrates. EMSA with (a) double-stranded linear DNA, (b) mismatch DNA, (c) gap DNA, (d) single-stranded DNA, (e) 3' overhang DNA and with (f) 5' overhang DNA. The DNA–protein complexes were resolved in 7% (w/v) non-denaturing polyacrylamide gels as described in Methods. MtbHU–DNA interaction The dissociation constant for the binding of 30 bp DNA was measured by surface plasmon resonance to be 6.4±0.4 nM, Table 2 . In addition, electrophoretic mobility shift assays (EMSA) demonstrated unequivocally that MtbHU could bind to a variety of DNA substrates, that is, those with gaps, overhangs and mismatches ( Fig. 2 , Supplementary Fig. 2c ; for the DNA sequences, see Supplementary Table 1 ). MtbHU–DNA complexes were detected with 30 bp DNA ( Fig. 2a ), with DNA containing mismatches ( Fig. 2b ), 1-nt gapped DNA ( Fig. 2c ) and DNA with 3' or 5'-overhangs ( Fig. 2e,f ). With the exception of the 30-mer single-strand DNA ( Fig. 2d ), the remaining showed stable complexes. When the genome compaction ability of MtbHU was tested by overexpressing the protein in M. smegmatis mc [2] cells, a highly condensed, dot-shaped nucleoid was observed, compared with the control cells that showed nucleoids of regular size and shape ( Fig. 3 and Supplementary Fig. 4a,b ). The protein colocalized with the condensed nucleoid (Methods; Supplementary Fig. 4c ), indicating the direct role of MtbHU in genome compaction. Table 2 Binding affinities for DNA, SD1 and SD4 binding to MtbHU. Full size table Figure 2: Binding of MtbHU to different DNA substrates. ( a – f ) Comparative EMSA showing the binding of increasing amounts of MtbHU to a fixed concentration of different DNA substrates. EMSA with ( a ) double-stranded linear DNA, ( b ) mismatch DNA, ( c ) gap DNA, ( d ) single-stranded DNA, ( e ) 3' overhang DNA and with ( f ) 5' overhang DNA. The DNA–protein complexes were resolved in 7% (w/v) non-denaturing polyacrylamide gels as described in Methods. 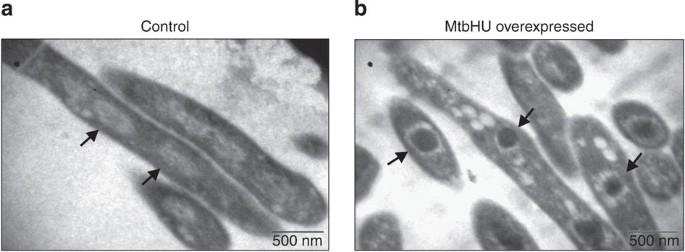Figure 3: Effect of MtbHU overexpression on nucleoid structure. Ultrastructure analysis ofM. smegmatiscells overexpressing MtbHU. (a) In the electron micrographs control cells show the regular bi-lobular nucleoid (arrows), whereas (b) the MtbHU-overexpressing cells have highly compact electron dense nucleoid (arrows). Scale bars, 0.5 μm. Full size image Figure 3: Effect of MtbHU overexpression on nucleoid structure. Ultrastructure analysis of M. smegmatis cells overexpressing MtbHU. ( a ) In the electron micrographs control cells show the regular bi-lobular nucleoid (arrows), whereas ( b ) the MtbHU-overexpressing cells have highly compact electron dense nucleoid (arrows). Scale bars, 0.5 μm. Full size image The higher resolution P2 1 structure (4PT4) was used for the modelling studies. The structurally rigid and flexible domains of MtbHU, as derived from the crystallographic and computational analyses, were defined as substructures/segments. These were then used as input for segmentation guided energy minimization and molecular dynamic simulations ( Supplementary Methods ) to construct a model for the MtbHU N –DNA complex ( Fig. 4 ). The protein–DNA interaction surface is primarily composed of positively charged residues (Lys3, Arg53, 55, 58, 61, 64, 80 and Lys86). Except for Lys3 in S1, the rest of the positively charged residues are located in S2 and they provide the key interactions for DNA binding. Upon DNA binding, the mobile loops (residues 61–66) from each protomer execute a pincer-like movement and hold the DNA by its minor groove in a vice-like grip. Pro63 in each protomer located at the tips of the loops intercalate between the base pairs of DNA minor groove, at sites that are 9 bp apart ( Fig. 5a ; site I), inducing a bend in the DNA. The importance of the residues located at the DNA-binding β-cleft, namely Arg55, 58 and 61, has also been reported for HU from Bacillus stearothermophilus [29] . In addition to the interactions with subdomain S2, interactions between DNA and the residues that connect S1 and S2, viz., residues 38–48 (refs 30 , 31 ), further stabilize the complex. A detailed account of MtbHU–DNA interactions is provided in Supplementary Table 2a and Supplementary Discussion . A comparative analysis of the MtbHU–DNA modelled structure with the co-crystal structure of Anabaena HU (1P71 and 1P51) [5] and Hbb, a homologue of HU from Borrelia burgdorferi (2NP2) [7] , is provided in Supplementary Table 2b . It is evident from the analyses that the key residues from the DNA-binding cleft, such as Arg53, 55, 58, 61, 64, 80 and Lys86, or their equivalent residues ( Supplementary Fig. 5 ) are involved in DNA interaction across species, Supplementary Table 2b . Further, the comparison reveals that while the 20-bp DNA in Anabena HU co-crystal structure involves residues primarily from the DNA-binding cleft, in case of longer DNA, the interactions span beyond the β-cleft, and include Lys11 and Ser59 in B. burgdorferi Hbb and their equivalents Lys3 and Gly46 in MtbHU ( Supplementary Table 2b ). Thus, a combination of electrostatic interactions involving a constellation of positively charged residues, networks of hydrogen bonds and minor groove intercalation aided by the inherent flexibility of MtbHU’s DNA-binding β-saddle contribute to its ability to bind and bend various DNA substrates. 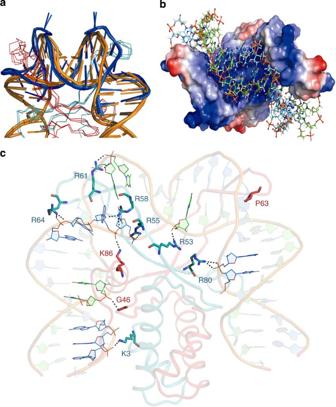Figure 4: MtbHU–DNA interaction. (a) Initial and final states of energy-minimized MtbHUNcomplexes with 20 bp DNA (in blue) and 30 bp DNA (in orange), are superimposed to display the flexible nature of MtbHU–DNA interaction. For clarity, the protein is shown as a backbone trace representation (protomer A: red, protomer B: teal), while DNA in cartoon. Light and dark blue coloured DNA represent the initial and final states of 20 bp oligo bound to MtbHUN; for the 30 bp DNA, the states are shown in light and dark orange respectively. (b) Charge complementarity in MtbHUN–DNA interaction:DNA backbone phosphates bind at the interface of S2 carrying positively charged Lys and Arg residues; colour codes corresponding to residue charges (blue: positive, red: negative). (c) MtbHUNside chain interacts with DNA, involving positive charge residues Lys3, Arg53, 55, 58, 61, 64, 80 and Lys86 from each protomer. For clarity, side chains of these residues are shown in stick representation and amino-acid residues in single letter codes. Pro63 approaches the DNA through minor groove intercalation. Figure 4: MtbHU–DNA interaction. ( a ) Initial and final states of energy-minimized MtbHU N complexes with 20 bp DNA (in blue) and 30 bp DNA (in orange), are superimposed to display the flexible nature of MtbHU–DNA interaction. For clarity, the protein is shown as a backbone trace representation (protomer A: red, protomer B: teal), while DNA in cartoon. Light and dark blue coloured DNA represent the initial and final states of 20 bp oligo bound to MtbHU N ; for the 30 bp DNA, the states are shown in light and dark orange respectively. ( b ) Charge complementarity in MtbHU N –DNA interaction:DNA backbone phosphates bind at the interface of S2 carrying positively charged Lys and Arg residues; colour codes corresponding to residue charges (blue: positive, red: negative). ( c ) MtbHU N side chain interacts with DNA, involving positive charge residues Lys3, Arg53, 55, 58, 61, 64, 80 and Lys86 from each protomer. For clarity, side chains of these residues are shown in stick representation and amino-acid residues in single letter codes. Pro63 approaches the DNA through minor groove intercalation. 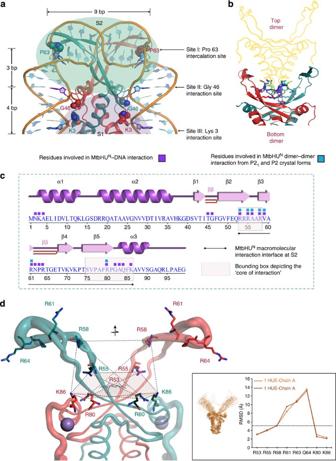Figure 5: Adaptive macromolecular interface at S2, common to both DNA binding and self-assembly. Residues involved in (a) DNA binding and (b) self-assembly are plotted onto a secondary structure representation of MtbHUNwith the help of purple and blue blocks, respectively, shown in (c). (d) Important residues such as Arg53, 55, 61, 64, 80 and Lys86 from each protomer are depicted in stick representation; mapped along with the structural dynamicity of the MtbHUNhomodimer, expressed through ‘B-factor putty’. The box marked with dotted lines depicts the ‘region of core interactions’ consisting of residues 53–58 and 75–86. The same is represented by the boxed region in (c). The ‘core region’ omits the DNA interacting residues Arg61, 64 and Pro63 from the highly mobile loops, and constitutes a smaller search space for inhibitor binding studies (Supplementary Fig. 7). The inset for (d) shows a comparison of structural dynamicity with the solution structure of HU fromB. stearothermophilus(PDB ID: 1HUE, ensemble structure in left, colour code: orange). In right, side-chain centroid r.m.s.d. (Supplementary Methods) shows residue 53, 55, 58, 80 and 86 of 1HUE to be ‘less’ mobile, similar to that observed for the core residues in MtbHU. Full size image Figure 5: Adaptive macromolecular interface at S2, common to both DNA binding and self-assembly. Residues involved in ( a ) DNA binding and ( b ) self-assembly are plotted onto a secondary structure representation of MtbHU N with the help of purple and blue blocks, respectively, shown in ( c ). ( d ) Important residues such as Arg53, 55, 61, 64, 80 and Lys86 from each protomer are depicted in stick representation; mapped along with the structural dynamicity of the MtbHU N homodimer, expressed through ‘B-factor putty’. The box marked with dotted lines depicts the ‘region of core interactions’ consisting of residues 53–58 and 75–86. The same is represented by the boxed region in ( c ). The ‘core region’ omits the DNA interacting residues Arg61, 64 and Pro63 from the highly mobile loops, and constitutes a smaller search space for inhibitor binding studies ( Supplementary Fig. 7 ). The inset for ( d ) shows a comparison of structural dynamicity with the solution structure of HU from B. stearothermophilus (PDB ID: 1HUE, ensemble structure in left, colour code: orange). In right, side-chain centroid r.m.s.d. ( Supplementary Methods ) shows residue 53, 55, 58, 80 and 86 of 1HUE to be ‘less’ mobile, similar to that observed for the core residues in MtbHU. Full size image Rationale for the design of MtbHU–DNA interaction inhibitor The large adaptive target site of DNA-binding β-saddle underscores the challenge of applying conventional structure-based design strategies to accurately identify inhibitors that are ‘drug-like’, in terms of molecular weight and specificity. In silico screening with property-based pre-filtering and GLIDE docking [32] , [33] (Methods) was performed to identify compounds that exhibited DNA mimicking interactions with the positively charged residues Arg53, Arg55, Arg58, Arg61, Arg64, Arg80 and Lys86. Initial screening yielded large polyanaionic inhibitors, such as suramin and its derivatives with molecular weight >1 kDa, which are likely to be non-specific. To obtain smaller molecules that can bind specifically to the β-saddle, a critical analysis of the binding site was undertaken. The packing observed in the crystal-polymorphs suggested that the DNA-binding surface of S2 can also act as a protein–protein interaction surface that facilitates self-assembly ( Fig. 5b , Supplementary Fig. 6 , Supplementary Tables 3–5 and Supplementary Discussion ). Comparison of binding site interactions with DNA, ligands and self led to the identification of an interaction core, located within the saddle of S2, made by residues Arg53, 55, 58, 80 and Lys86 ( Fig. 5c,d ). Screening for ligands that target this ‘core’ (details in Supplementary Fig. 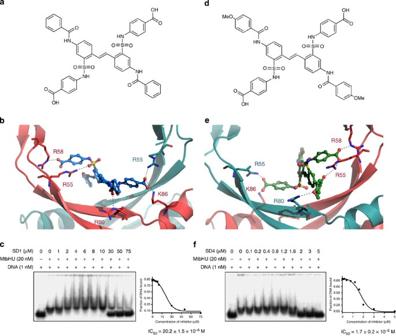Figure 6: Structure-based lead identification for the inhibition of MtbHU–DNA interaction. SD1 and SD4 screened using Virtual Screening Workflow (Schrödinger Discovery Tool). (a) SD1 (PubChem CID: 5821513), atrans-stilbene derivative. (b) Energy-minimized model of SD1 bound to the protein based on the GLIDE dock-pose. In the figure, hydrogen bond interactions between SD1 and the positively charged residues Arg55, 58, 80 and Lys86 of MtbHUNare shown. The same residues are also involved in electrostatic interactions, see text for details. (c) Inhibition of MtbHU–DNA binding by SD1 and its corresponding inhibition curve (inset, IC50value). (d) SD4, a methoxy derivative of SD1. (e) Energy-minimized model of SD4 bound to the protein based on the GLIDE dock-pose. In the figure, hydrogen bond interactions between SD4 and the positively charged residues Arg55, 58, 80 and Lys86 of MtbHUNare shown. The same residues are also involved in electrostatic interactions, see text for details. (f) Inhibition of MtbHU–DNA binding by SD4 and its corresponding inhibition curve (inset, IC50value). 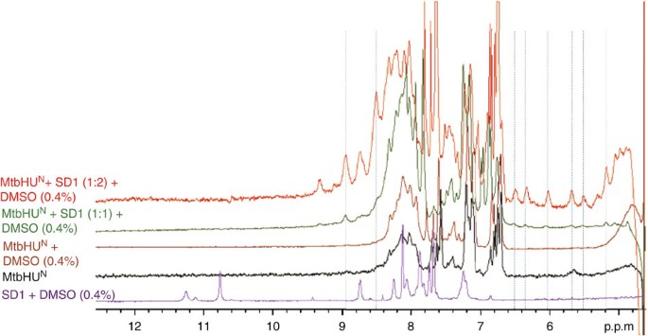Figure 7: SD1 induced changes in NMR spectra of MtHUN. The dotted lines indicate the resonance lines that are observed upon ligand binding. Line narrowing is clearly visible upon increasing the ligand concentration from a protein to ligand ratio of 1:1 (in green) and 1:2 (in red). The spectra of MtbHUNin the presence and absence of co-solvent (DMSO) and of SD1 in DMSO are shown in black, brown and purple respectively. 7 and Supplementary Table 6 ) identified a set of 36 compounds ( Supplementary Table 7 ). Next, EMSA was performed to test the screened compounds for the inhibition of MtbHU–DNA binding. Stilbene derivatives inhibit MtbHU and cell growth EMSA identified two trans -stilbene derivatives, 4, 4′-[(E)-ethene-1, 2-diylbis ({5[(phenylcarbonyl)amino]benzene-2,1-diyl}sulfonylimino)]dibenzoic acid and its methoxy derivative 4,4′-[1,2-ethenediylbis({5-[(4-methoxybenzoyl)amino]-2,1phenylene}sulfonylimino)]dibenzoic acid, referred to as SD1 ( Fig. 6a–c ) and SD4 ( Fig. 6d–f ) respectively, as the two most potent inhibitors. SD1 showed 50% inhibition (IC 50 ) of DNA binding at 20 μM concentration and SD4 showed an IC 50 of 1.7 μM. In case of SD4, one of the methoxy oxygens (absent in SD1; Fig. 6b ) showed an additional interaction with Arg80 from chain B of MtbHU N ( Fig. 6e ), presumably contributing to its higher potency. Further details of the binding site interactions of SD1 and SD4 are provided in Supplementary Fig. 8 . Both SD1 and SD4 showed intrinsic fluorescence, which increased when they bound MtbHU, due to the reduction of solvent quenching (Methods; Supplementary Fig. 9 ). The binding affinities of the compounds determined by fluorescence spectroscopy are listed in Table 2 . The minimal inhibitory concentrations (MIC) of SD1 and SD4 for Mtb H37Ra were determined by resazurin microtitre plate assay [34] (Methods). The MICs were found to be ~400 and 800 μM, respectively. Interestingly, the compound with lower binding affinity, that is, SD1 had a better MIC. Several factors could, in principle, contribute to the intra-cellular availability of the inhibitor, viz., permeability, solubility and stability. Of significance is the observation that the Mtb cells treated with the compound had a diffused nucleoid structure, distinct from that in the untreated cells (see next section). Figure 6: Structure-based lead identification for the inhibition of MtbHU–DNA interaction. SD1 and SD4 screened using Virtual Screening Workflow (Schrödinger Discovery Tool). ( a ) SD1 (PubChem CID: 5821513), a trans -stilbene derivative. ( b ) Energy-minimized model of SD1 bound to the protein based on the GLIDE dock-pose. In the figure, hydrogen bond interactions between SD1 and the positively charged residues Arg55, 58, 80 and Lys86 of MtbHU N are shown. The same residues are also involved in electrostatic interactions, see text for details. ( c ) Inhibition of MtbHU–DNA binding by SD1 and its corresponding inhibition curve (inset, IC 50 value). ( d ) SD4, a methoxy derivative of SD1. ( e ) Energy-minimized model of SD4 bound to the protein based on the GLIDE dock-pose. In the figure, hydrogen bond interactions between SD4 and the positively charged residues Arg55, 58, 80 and Lys86 of MtbHU N are shown. The same residues are also involved in electrostatic interactions, see text for details. ( f ) Inhibition of MtbHU–DNA binding by SD4 and its corresponding inhibition curve (inset, IC 50 value). Full size image Target specificity of SD1 That the compound binds to MtbHU N in solution was studied using NMR. Figure 7 shows a stacked plot representation of the one-dimensional NMR spectra of the MtbHU N as a function of SD1 concentration. Also shown in the figure are the spectra of MtbHU N and SD1, which serve as controls. The spectrum of MtbHU N shows broad resonances, suggesting that the molecule is undergoing either oligomerization, which would increase the effective molecular weight in solution, or intramolecular conformational exchange. Similar conformational fluctuations have been reported in case of other HUs [35] , [36] . Upon binding SD1, sets of sharp resonances were observed for the residues in the protein in the 8.5–9.5 p.p.m. and 5.2–6.5 p.p.m. regions. Alpha protons of residues in β-sheets of proteins generally appear in the latter region [37] . The compound SD1 has a pair of olefinic protons that resonate further downfield (~7.1 p.p.m.) and hence does not contribute to the spectrum in the 5.2–6.5 p.p.m. region ( Fig. 7 ). Further, the resonance lines in MtbHU N sharpen as a function of the concentration of the ligand SD1 (MtbHU N -SD1=1:1 in green and 1:2 in red; Fig. 7 ) in the above indicated regions of the spectrum. Comparison of the spectra of MtbHU N +SD1 with the spectrum of SD1 once again shows that the observed resonance lines are of protein origin. The line narrowing indicates that the rate of transition between conformational states migrates either into the fast exchange regime or the slow exchange regime, where the minor populations are below the detectable limit of the NMR methods applied here. Overall, the NMR study provided physical evidence of the SD1–MtbHU N interaction, although the exact binding site on the protein could not be revealed. Figure 7: SD1 induced changes in NMR spectra of MtHU N . The dotted lines indicate the resonance lines that are observed upon ligand binding. Line narrowing is clearly visible upon increasing the ligand concentration from a protein to ligand ratio of 1:1 (in green) and 1:2 (in red). The spectra of MtbHU N in the presence and absence of co-solvent (DMSO) and of SD1 in DMSO are shown in black, brown and purple respectively. Full size image In order to confirm the target site, alanine replacement mutations were carried out for the MtbHU residues that lie at the ‘core’ of the DNA-binding β-cleft. The mutation in Arg55, 58, 80 and Lys86 led to reduced binding of both the inhibitors and DNA ( Table 2 ; Supplementary Fig. 9 ). It may be noted that, in effect, each single point mutation is duplicated since functional HU is a homodimer. Each of the mutant proteins bound the stilbene derivatives and DNA with reduced affinity when compared to wild-type MtbHU ( Table 2 , Supplementary Fig. 9 ). All the mutants had lower affinity, indicating the specificity of these inhibitors for the DNA-binding β-saddle. Predictably, one of the compounds tested bound to both M. smegmatis and E. coli HU and inhibited their binding to DNA ( Supplementary Fig. 10a,b ). Inhibition of E. coli HU is to a lower extent, but importantly both M. smegmatis and E. coli growth was not affected by the inhibitor (see below). The specificity of the stilbene derivative to HU is verified by the observation that the inhibitor did not perturb the binding of DNA to other NAPs such as Lsr2 and H-NS (Rv3852) of Mtb or E. coli Fis ( Supplementary Fig. 10b ). That the molecule targets MtbHU in vivo , inhibits its DNA binding and disrupts nucleoid is substantiated by the following experiments. The MIC of SD1 for Mtb H37Ra cells in which the MtbHU was overexpressed was higher, suggesting a relation between the level of MtbHU expression and the inhibitory concentration of the compound ( Supplementary Fig. 11 and Supplementary Methods ). Although, DNA binding of HU from both E. coli and M. smegmatis were inhibited in vitro , treatment with SD1 in the concentration range of 3–1,600 μM did not cause growth inhibition of these bacteria. This is possibly due to non-essentiality of HU in these species and the presence of additional NAPs in their genomes with similar functions [38] , [39] . Importantly, a conditional knockdown strain of MtbHU, in which expression of HU can be downregulated, was constructed to validate its essentiality. The strain showed nucleoid de-compaction and compromised growth upon HU depletion ( Supplementary Fig. 12a–c ). Inhibitor-treated Mtb cells also showed diffused nucleoid structure ( Fig. 8a,b ). Expression analysis in the knockdown strain revealed reduced expression of a set of genes, whose expression is downregulated upon inhibitor treatment ( Supplementary Fig. 12d ). Similarly, Rv0559 was upregulated in both inhibitor-treated and the HU-depleted strain ( Supplementary Fig. 12d ). Thus, mutation studies, perturbation of nucleoid structure, cell growth inhibition and genetic knockdown together indicate target specificity of the molecule against MtbHU and selective killing of Mtb. 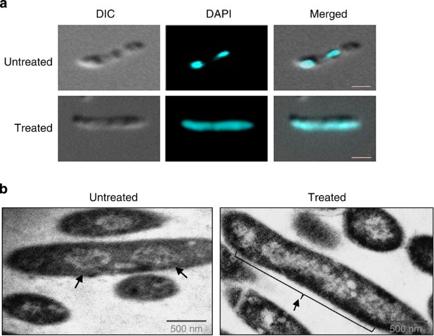Figure 8: Effect of SD1 treatment on nucleoid morphology of Mtb. (a) Fluorescent micrograph of Mtb cells showing DAPI-stained condensed nucleoid in untreated cells (top) and dispersed nucleoid (bottom) in SD1 treated cells. Scale bar, 1 μm. (b) Transmission electron micrographs of untreated Mtb cells (left) with confined bi-lobular nucleoid (arrows), and of SD1-treated cells (right) with nucleoid spread along the cell length displaying the lack of compactness. Scale bar, 0.5 μm. Figure 8: Effect of SD1 treatment on nucleoid morphology of Mtb. ( a ) Fluorescent micrograph of Mtb cells showing DAPI-stained condensed nucleoid in untreated cells (top) and dispersed nucleoid (bottom) in SD1 treated cells. Scale bar, 1 μm. ( b ) Transmission electron micrographs of untreated Mtb cells (left) with confined bi-lobular nucleoid (arrows), and of SD1-treated cells (right) with nucleoid spread along the cell length displaying the lack of compactness. Scale bar, 0.5 μm. Full size image A feature common to all NAPs is their ability to control genome architecture and influence various DNA transactions. HU is an essential NAP for Mtb function [19] , [20] . The critical importance of this NAP to Mtb survival prompted us to survey its function in the organism, achieved by selective inhibition of its DNA-binding properties. Crystal structures and computational analysis revealed the adaptive nature of HU’s DNA-binding β-saddle, which also engages in self-assembly. The residues in the β-saddle were resolved into two different regions, (i) the ‘core region’, which is located at the base of the saddle, responsible for docking with DNA or another HU dimer and (ii) the region corresponding to residues 61–66, which forms the highly mobile loop tips of DNA embracing β-arms, that is, the ‘dynamic rim region’. This rim region of each protomer facilitates DNA bending through conformational changes induced by DNA binding. Our study here elucidates that, to perturb MtbHU–DNA interaction, it is sufficient to target just the ‘core region’ ( Fig. 5 and Supplementary Fig. 7 ). Several lines of evidence indicate that such a strategy is not without merit. For instance, EMSA studies have demonstrated that the stilbene derivatives, identified using the above rationale, competitively inhibit HU binding to DNA. Site-directed mutation of residues at the core indicated that these residues are common to both DNA and inhibitor interactions. The solution NMR studies indeed show spectral changes originating from the protein, as a function of the concentration of SD1, implying the formation of MtbHU–inhibitor complex. Quantitative studies using fluorescence spectroscopy have yielded the binding affinities of the inhibitors for HU. In vivo studies have shown that the inhibitor affects nucleoid architecture in the cell and furthermore inhibits Mtb growth. Macromolecular interfaces, such as protein–DNA/protein–protein interactions sites, offer a rich landscape for the discovery of new-generation drugs. However, conventional drug development methods have generally shied away from this potentially important target because of ‘undesirable’ features like large binding site and the need for adaptive changes in conformation at the protein–ligand binding interface [21] , [40] , an issue that we have addressed in the present report. Perturbation of MtbHU–DNA binding, by targeting the ‘core region’, with SD1 and SD4 provides the first instance of medium to small molecular weight inhibitors of NAP, demonstrating that HU is ligandable. The structure-based studies along with the comparative analysis with other HUs suggest that the key residues from the DNA-binding cleft, such as Arg53, 55, 58, 61, 64, 80 and Lys86, or their equivalent residues ( Supplementary Fig. 5 and Supplementary Table 2b ), are involved in DNA interaction and are maintained across species. Further, analysis of the side chain r.m.s.d. ( Supplementary Methods ) based on the solution structure of HU from B. stearothermophilus (PDB ID: 1HUE) reveals residues 53, 55, 58, 80 and 86 to be the ‘less’ mobile ones, as seen for the core residues in MtbHU ( Fig. 5d ). Interestingly, the similarities continue to the analysis of crystal packing and unit cell dimensions of the HU from B. stearothermophilus ( Supplementary Table 5 ; PDB ID: 1HUU). Together, the observations suggest that the same rationale outlined here for developing inhibitors could be extended to other homologous protein targets with HU fold, harbouring the sequence pattern, prosite PS00045. The adverse effects of the inhibitors on nucleoid architecture and cell growth underscore HU as a target, at least in organisms such as Mtb, whose genome has a remarkable under-representation of NAPs [41] . Given the striking sequence conservation among HUs from different pathogenic mycobacterial species including M. leprae , M. bovis and other pathogenic actinobacteria, such as Nocardia , particularly at the N-terminal DNA-binding region ( Supplementary Fig. 1 ), we envision that the inhibitor design strategy outlined here can serve as a template to target the NAP in these organisms. Many NAPs, including HU, play a crucial role in the global regulation of transcription and various DNA transactions. Despite being a ‘hub point’ of cellular regulatory network, no inhibitor molecule has been reported so far to target this particular NAP, or, for that matter, any other NAP. SD1 is a new chemical probe developed to perturb HU–DNA interaction in Mtb. Thus, this ‘proof of principle’ study opens up avenues to monitor the role of the NAP in genome organization, gene expression and critical processes in different cellular contexts. The approach could provide an insight into HU-controlled regulons and contribute towards a better understanding of the role of HU in particular and other NAPs in general. Structure-based inhibition of an essential NAP described here could also form the basis for targeting other NAPs through novel inhibitor design. Cloning, overexpression and purification of MtbHU Rv2986c ( hupB ) was PCR-amplified from Mtb H37Ra genomic DNA using gene-specific forward and reverse primers containing the restriction enzyme sites Nde I and Eco RV, respectively ( Supplementary Table 1 ), cloned into E. coli expression vector pET20b to obtain pET20b- hupB . Same set of forward and reverse primers contained BamH I and Xba I restriction enzyme sites for cloning into mycobacterial expression vector pJAM2 to obtain pJAM2- hupB construct. The MtbHU N (residues 1–100) overexpression construct pET20b- hupB N was obtained by PCR-amplifying the gene segment with the same forward primer and internal reverse primer containing Xho I site ( Supplementary Table 1 ). The product was ligated into a pET20b vector to generate a C-terminal histidine tag-containing construct. The clones were confirmed by DNA sequencing. E. coli BL21 (DE3) pLysS cells were transformed with pET20b- hupB or pET20b- hupB N and the overexpression of the recombinant proteins was obtained by addition of 0.3 mM IPTG for 3 h. E. coli cells overexpressing MtbHU were lysed by sonication in buffer A (50 mM sodium phosphate, pH 7.4), 100 mM KCl, 1 mM EDTA and 0.1 mM phenylmethanesulfonyl fluoride (PMSF) and centrifuged at 13,000 r.p.m. at 4 °C for 20 min. After raising salt concentration of the supernatant to 800 mM with KCl and 0.8% polyethylenimine (v/v) precipitation, the supernatant was subjected to ammonium sulphate fractionation. The pellet (40–65% saturation) was resuspended in buffer A and loaded onto pre-equilibrated phosphocellulose column. The protein was eluted with 100–1,500 mM linear KCl gradient. MtbHU containing fractions were pooled and dialyzed against buffer B (10 mM Tris–HCl (pH 7.5), 250 mM KCl, 5% glycerol (v/v), 0.1 mM PMSF), passed through SP sepharose and heparin sepharose successively, and eluted with a linear gradient of 250–1,000 mM KCl. The purified protein was dialysed against buffer B and the concentration of the protein was estimated by the method of Bradford. The MtbHU N -overexpressing cells were lysed in buffer C (50 mM sodium phosphate (pH 7.4), 100 mM NaCl and 0.1 mM PMSF) and centrifuged at 13,000 r.p.m. at 4 °C for 20 min. The supernatant was loaded on to Ni-NTA column in the presence of 10 mM imidazole and eluted with 500 mM imidazole containing buffer C. The protein-containing fractions were pooled and dialyzed against buffer C, passed through SP sepharose and eluted with a linear gradient of 100–1,000 mM NaCl. The purity of the proteins was ascertained by resolving in 15% SDS-polyacrylamide gels. For crystallization the proteins were dialysed against a buffer containing 10 mM Tris–HCl (pH 7.5) and 50 mM KCl and concentrated using 10-kDa centricons. The crystallization trials were performed with both MtbHU N and the full-length MtbHU. However, even with the full-length protein, the crystals obtained (P2 1 ) were devoid of the C-terminal domain containing the low-complexity repeat region [6] . Glutaraldehyde crosslinking MtbHU protein (2 μg) was incubated at 30 °C for 10 min in 40 mM HEPES (pH 7.4) and 50 mM KCl. Glutaraldehyde was added at increasing concentrations (0.001–0.05% (v/v)) and incubated for an additional 2 min at 30 °C. The reactions were terminated with 200 mM Tris–HCl (pH 7.5) for 5 min at 4 °C and resolved in 12% SDS–PAGE at 80 V for 3 h followed by silver staining. Crystallization and data collection Plate–shaped crystals were obtained by hanging drop vapour diffusion method, in two conditions, containing (i) 0.1 M Tris–HCl (pH 8.2), 3 M sodium formate, and (ii) 0.1 M Tris–HCl (pH 6.7), 3.5 M sodium formate, with 10 mM MnCl 2 at HU concentration of 14 mg ml −1 (at 293 K). Diffraction data were collected on beamline X29A (X-ray wavelength 0.979 Å), at the National Synchrotron Light Source in Brookhaven National laboratory. Crystals grown in the first condition diffracted to 2.04 Å resolution, whereas crystals from condition (ii) diffracted to 2.48 Å (at 100 K). The data sets were processed using HKL-2000 suite [42] . Crystals from the two variants of sodium formate condition belonged to monoclinic P2 1 and P2 space groups respectively, each containing two protomers of MtbHU N per asymmetric unit. Structure determination The structure of N-terminal of HU dimer from Mtb was determined by molecular replacement (MR) method using the programme PHASER [43] . At first, MR was performed with the diffraction data obtained from the P2 1 crystals. The initial solution was subjected to several stages of model building with careful inspection of map using the COOT programme [44] and refinement using REFMAC5 (refs 45 , 46 ). The model bias was removed using composite omit map and the structure was validated through PROCHEK [47] analysis. Refined coordinates from P2 1 data set were used as search models during the MR of the P2 data set. See Table 1 and Supplementary Methods for additional details. Electrophoretic mobility shift assay The sequences of the oligonucleotides used in EMSA are given in Supplementary Table 1 . The oligonucleotide graA was 5′ end labelled with [γ- 32 P] ATP by T4 polynucleotide kinase. Double-stranded DNA substrate (30 bp) was prepared by annealing oligonucleotides graA and graB, 3′-overhang substrate by annealing graA and graD, gapped DNA by annealing graA, graC and graD. Mismatched DNA was prepared by annealing graA and graM. The DNA substrates (1 nM each) were incubated with increasing concentration of MtbHU on ice for 20 min in binding buffer containing 10 mM HEPES (pH 7.4) and 50 mM KCl. The products were electrophoresed in 7% (w/v) non-denaturing polyacrylamide gels (39:1 acrylamide:bisacrylamide) in TBE (45 mM Tris−borate (pH 8.3) and 1 mM EDTA) and documented by Phosphorimager (Fujifilm). All the test compounds (Chembridge) were dissolved in DMSO. MtbHU and end-labelled 30-bp double-stranded DNA were pre-incubated on ice. Different concentrations of the compounds were added to the DNA–protein complex, incubated for 5 min and analysed in 7% (w/v) non-denaturing polyacrylamide gels as described above. Inhibition curves and IC 50 values were determined using GraphPad Prism 5 software. Preparation of compound library and docking Structures of compounds were downloaded from the ZINC database [48] , Pubchem and NCI’s chemical library compilation (downloaded from the web site ( http://cactus.nci.nih.gov/ncidb2/chem_www.html ) and processed with LigPrep software (available from Schrödinger, Portland, OR, USA). Successive steps of virtual screening protocol (Virtual Screening Workflow, part of the Schrödinger First Discovery Suite) were applied to this filtered subset of ligands to screen for the compounds with best potential to bind to MtbHU’s DNA-binding cleft. First, the ligands were treated with the ligprep module of Schrödinger Discovery Tool to remove counter ions, adjust charge states and generate tautomers wherever applicable. The b min module was used to generate energy-minimized structure for all of the compounds and high energy or strained geometry states were filtered. The final subset of filtered and prepared ligands was stored as a local ligand database. To prepare the receptor for docking, hydrogen atoms were added to the MtbHU N Structure (Protein Data Bank code 4PT4), which was then energy minimized using Protein Preparation Wizard (Schrödinger Discovery Tool). Docking was performed using virtual screening workflow of GLIDE, where molecules sorted by HTVS (high-throughput virtual screening) Glide were subjected to docking with ‘standard Precision’ GLIDE (SP Glide). The compounds with a SP Glide score better than −5 were subjected again to docking analysis through ‘extra-precision’ mode of GLIDE (XP Glide), which exacts severe penalties for complexes that violate established principles, such as that charged and strongly polar groups be adequately exposed to solvent [49] . H-bonding constrains were defined using the basic residues present at the DNA-binding cleft of MtbHU, namely Arg53, 55, 58, 61, 64, 80 and Lys86, to ensure that the final selection of molecules are screened for interactions with at least some of these residues. This strategy was selectively modified during the second stage of screening for smaller inhibitors following the identification of interaction core. The ‘enclosing box’ of docking grid for Stage II was generated using ‘centroid of selected residues’ option of GLIDE receptor grid generation module. Residues used for the enclosing box were Arg53, 55, 58, 80 and Lys86, where the ligand diameter midpoint box was calibrated to encompass residue 53, 55, 80 and 86 ( Supplementary Fig. 7 and Supplementary Table 6 ). At the end of the final XP Glide run, ligand poses and the conformations of the interacting sets of protein residues were post optimized with the help of Prime MM-GBSA module from Schrödinger Discovery Tools. The final screened compounds were scrutinized in their various binding poses to choose for molecules with most desirable sets of interactions using Glide XP Pose visualizer (Schrödinger Discovery Tool). To provide a refined model addressing the side chain flexibility of the interacting arginines and lysines at the binding site, HU-ligand docked complexes for SD1 and SD4 were further subjected to energy minimization, allowing side chains of the interacting residues to attain optimum conformation. Site-directed mutagenesis MtbHU mutants were generated by site-directed mutagenesis using the megaprimer inverse PCR method [50] . The oligonucleotides used in this study are listed in Supplementary Table 1 . Expression plasmid pET20b- hupB encoding the WT hupB gene was used as a template. Oligonucleotide primers carrying the respective amino acid codon substitutions were used for mutagenesis. After confirming the mutation by sequencing, the mutant proteins were expressed in E. coli BL21 (DE3) pLysS as described above. The mutant proteins were purified following the protocol used for MtbHU. Surface plasmon resonance spectroscopy The 30-bp double-stranded DNA ( Supplementary Table 1 , gra A and gra B) was biotin-labelled and immobilized onto an SA sensorchip (BIAcore 3000 system, GE Healthcare). The different concentrations of wild type and mutant proteins were injected in HBS (10 mM HEPES (pH 7.4), 250 mM NaCl, 3 mM EDTA and 0.005% (v/v) polysorbate 20) at a flow rate of 20 μl min −1 . Binding response was measured for 120 s after the end of the injection. Following each injection cycle, chip surfaces were regenerated with a short injection of 25 mM NaOH. Obtained sensorgrams were processed by BIAevaluation software (GE Healthcare). The kinetic parameters of protein–DNA interaction were analysed as described [51] . The steady-state binding constants were determined by fitting the data to 1:1 Langmuir isotherm. Fluorescent spectroscopy The affinities of the inhibitors binding to MtbHU were determined by fluorescent spectroscopy. The SD1 and SD4 showed intrinsic fluorescence ( λ excitation =315 nm and λ emission =420 nm). Fluorescence intensity of the compounds increased upon binding to protein. The fluorescence of SD1 was measured in phosphate buffer saline (PBS) at pH 7.5. For SD4, the measurement was carried out in PBS containing 10 mM Na 2 CO 3 at pH 8.5, since SD4 showed better solubility at higher pH. However, for the DNA or for a given inhibitor (SD1 or SD4), all the experiments with native protein and mutants of MtbHU were carried out under identical buffer and pH conditions, establishing relative affinities of the HU and its mutant. To determine the binding affinities of the compounds, 0.2 μM of each compound was incubated separately with increasing concentrations of wild type or mutant MtbHU proteins at 25 °C. The change in fluorescence intensity was measured using Shimadzu RF-5301 PC. The dissociation constant ( K d ) was calculated by plotting fractional saturation against concentrations of protein in nonlinear regression analysis [52] . Proton NMR spectroscopy Proton NMR spectra of MtbHU N alone and its complexes with SD1 were acquired on a 600-MHz Agilent NMR spectrometer, using a triple resonance (IDTRPFG) probe fitted with a single ( z axis) pulsed field gradient accessory. Samples of MtbHU N (400 μM) for NMR were prepared in 10 mM phosphate buffer (pH 7.5) containing 100 mM NaCl, 0.4% d 6 -DMSO, 90% H 2 O and 10% D 2 O. The protein–inhibitor complex was formed by gradual mixing of MtbHU N with SD1 in 1:1 or 1:2 molar ratios in a dilute solution. The complex was allowed to form for 30 min at 25 °C and the protein was concentrated to a final concentration of 400 μM. Proton spectra were collected at 25 °C, and sampled over a spectral width of 10,000 Hz. An interscan delay of 1 s was introduced between successive transients. Each spectrum was signal averaged over 1,024 transients. Inhibition of Mtb growth Inhibition of Mtb H37Ra cell growth was assessed by resazurin microtitre plate assay [34] . Briefly, 100 μl of Middlebrook 7H9 broth (with 1% albumin dextrose catalase (ADC), 0.05% Tween 80 and 0.01% SDS) containing varying concentrations (3–1,600 μM) of SD1 or SD4 were dispensed in each well of a 96-well plate. Bacterial suspension equivalent in turbidity to that of no. 1 McFarland standard was diluted 1:20 in 7H9 broth; a 100-μl inoculum was inoculated in each well. Plates were sealed and incubated at 37 °C for 2 weeks. Resazurin solution (25 μl; 0.02%) was added to each well and incubated for 24 h. A change in colour from blue to pink indicated the growth of bacteria, and the MIC was read as the minimum concentration of the inhibitor that prevented the colour change in resazurin solution. Fluorescence microscopy and transmission electron microscopy The pJAM- hupB plasmid or pJAM2 vector was transformed into M. smegmatis mc 2 cells. The colonies were grown in Middlebrook 7H9 broth at 37 °C till OD 600 0.6 and induced with 2% (w/v) acetamide for 6 h. Mtb H37Ra cells were grown in Middlebrook 7H9 broth (containing 1% ADC, 0.05% Tween 80 and 0.01% SDS) till OD 600 0.6, treated with SD1 (200 μM) and incubated for 12 h at 37 °C. Cells were fixed overnight in 0.1 M sodium cacodylate (pH 7.5), 2% formaldehyde and 2.5% glutaraldehyde at 4 °C. For fluorescence microscopy, cells were stained with 4', 6-diamidino-2-phenylindole (DAPI) 0.1 μg ml −1 and images were acquired using AxioVs 40V.4.8.2.0 software on an epifluorescence microscope (Axio Imager M1) equipped with a × 100 1.4 numerical aperture oil differential interference objective and AxioCamMRm camera (Carl Zeiss, Inc.). Capture times and adjustments were similar for images mounted together. Fixed cells were processed for transmission electron microscopy analysis as described [53] . Briefly, cells were fixed with 0.1 M sodium cacodylate (pH 7.5), with 2% OsO 4 for 2 h and treated with 2% uranyl acetate for 1 h at RT. Cells were dehydrated with graded ethanol and embedded in Spurr resin. Sections of 50–70 nm thickness were stained with 1% uranyl acetate followed by lead citrate and visualized in JEOL 1200 transmission electron microscope equipped with a field emission gun electron source, operating at 80 kV. Image brightness and contrast were adjusted uniformly for all the images using Photoshop 7. Immunofluorescence microscopy Immunofluorescence microscopy was carried out as described in ref. 54 , with minor modifications. Briefly, MtbHU overexpressing M. smegmatis cells were fixed with 2% glutaraldehyde and 4% para-formaldehyde for 2 h, followed by several washes in PBS (pH 7.4). After permeabilization with lysozyme (2 mg ml −1 , 30 min, 37 °C) and triton X-100 (0.1%, 5 min, RT) cells were mounted onto poly-l-lysine-coated 12-well glass slides and blocked with PBS containing 0.05% Tween 20, 2% bovine serum albumin for 90 min. Affinity-purified mice anti-MtbHU antibodies (1:500) were applied overnight at 4 °C and goat anti-mouse secondary antibody FITC conjugate (1:400; GE Healthcare) was applied for 90 min. Cells were stained with DAPI (0.1 μg ml −1 ). Images were acquired using Axio Imager M1 microscope (Carl Zeiss, Inc.) as described above. Capture times and adjustments were similar for images mounted together. Generation of MtbHU conditional knockdown strain The hupB conditional knockdown strain of Mtb H37Ra was generated using TetR/Pip OFF system [55] . Briefly, a 250-bp region (−50 to +200 with respect to start codon) of hupB gene was amplified using specific primers (MtbHU-CK Frd and Rev, Supplementary Table 1 ) and cloned into Nsi I and Pvu II sites of pFRA50 to generate pFRA50-HU plasmid. To construct the promoter replaced strain, the pFRA50-HU was electroporated into Mtb H37Ra cells and the replacement was confirmed by PCR. The regulatory circuit containing pFRA42B [55] plasmid was electroporated into the promoter replaced strain to yield a conditional mutant of MtbHU (HU-CK). The HU-CK strain was grown on 7H9 broth (containing 1% ADC, 0.05% Tween 80 and 50 μg ml −1 hygromycin and 20 μg ml −1 streptomycin) at 37 °C till 0.5 OD and treated with 200 ng ml −1 anhydrotetracycline. The cell density was monitored at fixed time intervals. The depletion of MtbHU expression in mutant strain in the presence of anhydrotetracycline was confirmed by western blot analysis using affinity-purified anti-MtbHU polyclonal antibodies (1:5,000) ( Supplementary Methods ). Accession codes: Coordinates for MtbHU N in P2 1 and P2 crystal forms have been deposited in the RCSB Protein Data Bank under accession codes 4PT4 and 4DKY respectively. How to cite this article: Bhowmick, T. et al. Targeting Mycobacterium tuberculosis nucleoid-associated protein HU with structure-based inhibitors. Nat. Commun. 5:4124 doi: 10.1038/ncomms5124 (2014).